Epistasis and natural selection shape the mutational architecture of complex traits The evolutionary trajectories of complex traits are constrained by levels of genetic variation as well as genetic correlations among traits. As the ultimate source of all genetic variation is mutation, the distribution of mutations entering populations profoundly affects standing variation and genetic correlations. Here we use an individual-based simulation model to investigate how natural selection and gene interactions (that is, epistasis) shape the evolution of mutational processes affecting complex traits. We find that the presence of epistasis allows natural selection to mould the distribution of mutations, such that mutational effects align with the selection surface. Consequently, novel mutations tend to be more compatible with the current forces of selection acting on the population. These results suggest that in many cases mutational effects should be seen as an outcome of natural selection rather than as an unbiased source of genetic variation that is independent of other evolutionary processes. The relationship between the genotype and the phenotype, sometimes called the genotype–phenotype map, has taken centre stage in the study of complex traits for very good reasons [1] , [2] . For instance, many important human disorders, such as susceptibility to heart disease or Alzheimer’s disease, are determined by numerous genetic loci as well as environmental effects, thrusting these traits directly into the realm of quantitative genetics [3] , [4] . An understanding of how genes and the environment conspire to shape these traits might lead to better screening and treatment options. The complexity of the problem calls for an approach based on correlations of genetic variants with trait values, either in the context of genome-wide association studies or quantitative trait locus mapping [5] , [6] , but these approaches typically identify genetic loci that explain only a small fraction of the genetic variance in these sorts of complex traits [7] . This insufficiency problem has led to a widespread appreciation that interactions among genes, a phenomenon called epistasis in the quantitative genetics literature, could make a substantial contribution to the genetic variation in complex traits [5] , [6] , [7] , [8] , [9] , although the matter is still hotly debated [10] , [11] , [12] . An added wrinkle to these considerations is that traits do not exist in isolation from other traits. Individuals who express one trait, such as hypertension, may display a tendency to express other traits, such as diabetes [13] . In other words, different traits can be genetically correlated, and from an evolutionary standpoint we would like to understand how such genetic correlations arise and constrain population-level processes [14] . Genetic correlations can arise from a number of factors, and chief among them are natural selection and mutation [15] , [16] . If certain trait combinations confer a fitness advantage relative to others, then the variants that work well in combination will tend to be inherited together due to the increased fitness of their bearers [17] . From a mutation standpoint, if a mutation that affects one trait in a positive fashion also affects a second trait in a similar direction due to pleiotropy, then these new mutations will contribute to a genetic correlation between traits. This source of genetic correlations can be very strong indeed [18] , [19] , [20] . Given the central role of this ‘mutational architecture’ in the evolution of complex traits and the apparent importance of epistasis as revealed by studies of quantitative trait loci [9] , [21] , [22] , [23] , [24] , [25] , our goal in the present study is to investigate how epistasis influences the spectrum of mutations entering populations and how the evolution of mutational effects in turn constrains the genetic architecture of complex traits at the population level. Our results show that epistasis allows the mutational architecture of the multivariate phenotype to be shaped by natural selection and that the evolution of the mutational architecture in turn affects standing levels of genetic variance and the ability of a population to respond to selection. The epistasis model We model epistasis using an individual-based Monte Carlo approach to simulate a population of N individuals, each of which has a two-trait phenotype determined by both genetic and environmental effects. The genetic effects arise from a suite of n loci, each of which is pleiotropic and potentially epistatic. Epistasis is included using the multilinear approach [26] , [27] , [28] , which has been employed extensively to study the effects of epistasis on a single-trait phenotype [29] , [30] , [31] . Our implementation allows pairwise interactions among all loci. As the loci are pleiotropic, the epistatic effects can occur within or between trait effects. Our model accommodates both types of epistasis. An individual’s phenotype is determined by the sum of additive effects and epistatic terms (see Methods), plus an environmental effect drawn from a normal distribution with a mean of zero and variance of one. The life cycle consists of (1) random mating, (2) production of offspring, including mutation and recombination, (3) natural selection specified by a bivariate Gaussian individual selection surface (summarized by the ω -matrix) and (4) population regulation (see Methods for more details). 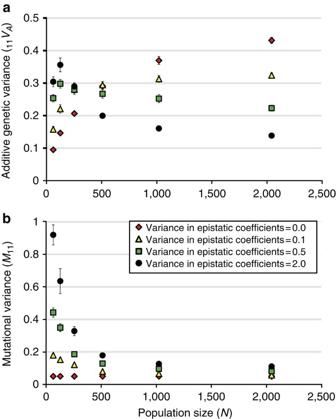Figure 1: The additive genetic variance and the mutational variance of a trait evolve as a function of underlying levels of epistasis. These simulation results were produced using our core set of parameters, except we imposed correlational selection,rω=0.9, and varied the population size from 64 to 2,048 across different runs. The top panel (a) shows the relationship between the equilibrium additive genetic variance for trait one and the population size. In a strictly additive model, larger populations maintain larger amounts of additive genetic variance (red diamonds), but with moderate-to-strong epistasis (green squares, closed circles) the pattern is reversed (with the exception of the smallest populations). The bottom panel (b) reveals the cause of this reversal. In an additive model, the mutational variance has no way to evolve, so small populations have the same equilibrium mutational variance as large populations (red diamonds). In the presence of epistasis, however, smaller populations evolve larger mutational variances than large populations (triangles, squares, circles), and these larger mutational variances in small populations contribute to a greater level of standing genetic variance, except when the effects of genetic drift are extremely strong (that is, whenN=64). In (a) and (b), error bars show one s.e.m. across 20 independent simulation runs; if error bars are not visible, then they are smaller than the symbol. We start with a core set of parameter values ( Table 1 ) and vary numerous combinations of parameters to investigate the evolution of the genetic variance and mutational architecture under a wide range of biologically plausible conditions. For each combination of parameters, we run the simulation for 5,000 initial generations to reach a balance between selection, mutation and genetic drift. These initial generations are followed by 5,000 experimental generations, during which we calculate variables of interest (see Methods). For each parameter combination, we conduct 20 independent runs of the complete simulation, including the 5,000 initial and 5,000 experimental generations. We average values of interest across these 20 independent runs. Our main variables of interest in the present model are the mutational variances ( M 11 and M 22 ) and mutational correlation ( r M ), which together describe the distribution of the phenotypic effects of new mutations entering the population and can be thought of as the mutational architecture of the two-trait phenotype, which we will also refer to as the M -matrix. We are also interested in the variables describing the distribution of genetic variation in the population, including the total genetic variances and covariance ( 11 V G , 22 V G and 12 V G ), the additive genetic variances and covariance ( 11 V A , 22 V A and 12 V A ), and the epistatic genetic variances and covariance ( 11 V AA , 22 V AA and 12 V AA ). The additive genetic variances and covariances determine the response of the population mean to selection, and are often organized into a matrix known as the G -matrix. Table 1 Key parameters and core parameter values for the multilivariate epistasis model. Full size table The evolution of the genetic variance and mutation matrix Several key results emerge from our analysis. The first major result is that epistasis affects the evolution of the genetic and mutational architecture of quantitative traits under a very wide range of parameter combinations. 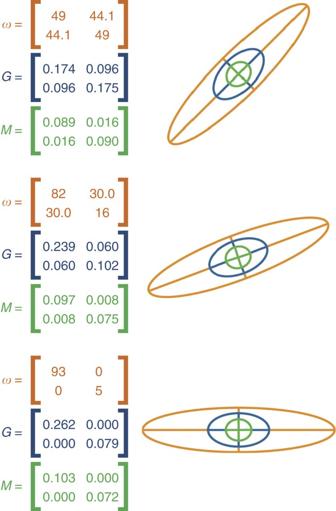Figure 2: Triple alignment of natural selection, genetic variation and mutation. Epistasis promotes alignment of the individual selection surface (theω-matrix), the additive genetic architecture (theG-matrix) and the mutational architecture (theM-matrix) of a two-trait phenotype. The actual matrices are shown to the left, and graphical depictions of the overlapping matrices are shown to the right. These results are from simulations using our core parameter set, except that population size is 4,096 and the individual selection surface (described byω) is held at a constant shape but oriented with its long axis turned in a different direction in phenotypic space for different simulation runs (but note that within a run the individual selection surface is always constant). The ellipses are 95-percent confidence ellipses, and the angle of the long axis of each ellipse is given by the leading eigenvector of the corresponding matrix (green forM, blue forGand orange forω) in a plot with trait one on thexaxis and trait two on theyaxis. Theω-matrix is not drawn to scale, but its orientation and proportions are correct. As the selection surface rotates, both theG-matrix and theM-matrix evolve to align with the selection surface in phenotypic space. This alignment result is extremely general and it occurs under almost all investigated parameter combinations. In particular, the mutational variances (that is, measures of the absolute size of the phenotypic effects of new mutations entering populations) of the quantitative trait loci show apparently adaptive changes in response to selection when epistasis is present ( Table 2 ), and these changes in mutational variances carry implications for the standing levels of genetic variance. 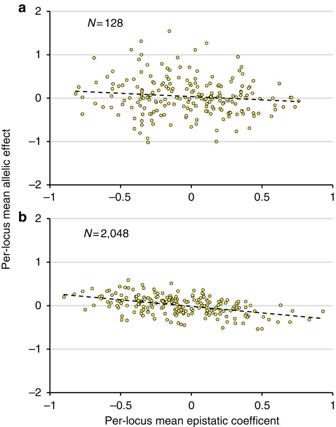Figure 3: Epistasis allows the mutational variance to evolve as function of population size. The average allelic effect can evolve to be correlated with the average epistatic coefficient, and the strength of this relationship varies with population size. These data are from 20 independent simulation runs using our core parameter set, except with only 10 quantitative trait loci. In addition, we allow only within-trait epistasis affecting trait one and no epistasis involving trait two, with population sizes of (a)N=128 and (b)N=2,048. Each point represents a single quantitative trait locus. Thexaxis shows the magnitude of epistasis (mean epistatic effect of a locus, averaged across all of its epistatic coefficients), and theyaxis presents the mean allelic effect (or reference effect) of alleles at the corresponding locus, averaged across all alleles segregating at the locus. In small populations, large mutational variances are maintained by the evolution of a large range in allelic effects; we see a slightly negative but non-significant relationship between epistatic coefficients and allelic effects (linear regression,N=200,R2=0.01,P=0.09). In large populations (b), which evolve lower mutational variances than small populations, we see a much smaller range in allelic effects and these effects show a strong negative relationship with the mean epistatic coefficients across loci (linear regression,N=200,R2=0.22,P<<0.0001). Thus, the allelic effects of a particular locus tend to evolve values that are largely counteracted by the epistatic effects of the locus in question. This figure is concerned with the evolution of the mutational variance, but a similar effect explains the evolution of mutational covariances. One striking result is that the magnitude of mutational variances is negatively related to population size ( Table 3 ). Table 2 The effects of the epistatic parameter variances on the genetic variance and the M -matrix. Full size table Table 3 The effects of population size on the evolution of the genetic variance and the M -matrix. Full size table The evolution of the mutational variances has a profound effect on the standing levels of genetic variation in our simulated populations. For instance, in a strictly additive model, mutational variances cannot evolve, and larger populations tend to harbour greater amounts of genetic variance compared with smaller populations due to reduced losses of variation because of a less-important role of genetic drift in the large populations ( Fig. 1 ). In the presence of epistasis, however, the situation changes dramatically. Smaller populations evolve larger mutational variances, and this pattern becomes more pronounced as the average absolute values of epistatic parameters increase ( Fig. 1 ; Table 2 ). These larger mutational variances increase the amount of genetic variance introduced by mutation each generation, which in turn increases the standing level of genetic variation. For moderately strong epistasis (that is, epistatic parameter variance, ), this increase in the mutational variance results in a tendency for larger populations to harbour less additive genetic variance than their smaller counterparts ( Fig. 1 ; Table 3 ). However, when populations become exceptionally small, the variance-reducing effects of drift become strong enough to overcome the increase in mutational variances, resulting in a non-monotonic relationship between population size and additive genetic variance under moderate to strong epistasis ( Fig. 1 ). Thus, the evolution of the mutational variance, as a consequence of evolving epistatic effects, has important implications at the population level in terms of standing levels of genetic variation. Figure 1: The additive genetic variance and the mutational variance of a trait evolve as a function of underlying levels of epistasis. These simulation results were produced using our core set of parameters, except we imposed correlational selection, r ω =0.9, and varied the population size from 64 to 2,048 across different runs. The top panel ( a ) shows the relationship between the equilibrium additive genetic variance for trait one and the population size. In a strictly additive model, larger populations maintain larger amounts of additive genetic variance (red diamonds), but with moderate-to-strong epistasis (green squares, closed circles) the pattern is reversed (with the exception of the smallest populations). The bottom panel ( b ) reveals the cause of this reversal. In an additive model, the mutational variance has no way to evolve, so small populations have the same equilibrium mutational variance as large populations (red diamonds). In the presence of epistasis, however, smaller populations evolve larger mutational variances than large populations (triangles, squares, circles), and these larger mutational variances in small populations contribute to a greater level of standing genetic variance, except when the effects of genetic drift are extremely strong (that is, when N =64). In ( a ) and ( b ), error bars show one s.e.m. across 20 independent simulation runs; if error bars are not visible, then they are smaller than the symbol. Full size image Triple alignment Our second major result is that the mutational covariance evolves in a way that causes adaptive alignment with the individual selection surface. If selection favors certain combinations of traits, then the presence of epistasis allows the mutational architecture to evolve in a way that new mutations tend to reinforce these favourable trait combinations. This alignment result is very general, and it occurs under almost all investigated parameter combinations, as evidenced by the evolution of a positive mutational correlation whenever we impose correlational selection ( Tables 2 and 3 ). We investigate the veracity of the alignment between the individual selection surface (the ω -matrix), the additive genetic architecture (the G -matrix) and the mutational architecture (the M -matrix), by conducting simulation runs involving selection surfaces oriented differently in phenotypic space, but otherwise of identical shape, and tracking the evolutionary responses of the G- matrix and M- matrix. When we perform this exercise, we find remarkable alignment between the ω -matrix, the G -matrix and the M -matrix ( Fig. 2 ). Under our parameter combinations, the elongate selection surface results in a somewhat less-elongate G -matrix, and in turn an even less-eccentric M -matrix, but the leading eigenvectors of all three matrices align almost perfectly in phenotypic space. These aligned M -matrices tend to remain stable within a run, and while different runs sometimes produce quantitatively different M -matrices, nearly all of them evolve toward alignment with the selection surface ( Supplementary Table 1 ). Figure 2 shows results from a large population ( N =4,096), but this sort of triple alignment also occurs in much smaller populations ( Supplementary Table 2 ), even though the alignment is disrupted somewhat in smaller populations by the operation of genetic drift. Figure 2: Triple alignment of natural selection, genetic variation and mutation. Epistasis promotes alignment of the individual selection surface (the ω -matrix), the additive genetic architecture (the G -matrix) and the mutational architecture (the M -matrix) of a two-trait phenotype. The actual matrices are shown to the left, and graphical depictions of the overlapping matrices are shown to the right. These results are from simulations using our core parameter set, except that population size is 4,096 and the individual selection surface (described by ω ) is held at a constant shape but oriented with its long axis turned in a different direction in phenotypic space for different simulation runs (but note that within a run the individual selection surface is always constant). The ellipses are 95-percent confidence ellipses, and the angle of the long axis of each ellipse is given by the leading eigenvector of the corresponding matrix (green for M , blue for G and orange for ω ) in a plot with trait one on the x axis and trait two on the y axis. The ω -matrix is not drawn to scale, but its orientation and proportions are correct. As the selection surface rotates, both the G -matrix and the M -matrix evolve to align with the selection surface in phenotypic space. This alignment result is extremely general and it occurs under almost all investigated parameter combinations. Full size image The evolution of larger mutational variances in small populations can be understood by considering the relationship between average allelic effects at the quantitative trait loci and the average epistatic coefficients for each locus. As the epistatic coefficients are parameters in the multilinear model, they do not change during a given simulation run (see Methods). Rather, epistatic contributions, and hence genotypic values, evolve as the allelic effects of individual loci change over evolutionary time. Loci with favourable epistatic coefficients can evolve larger allelic effects that enhance their epistatic effects. Alternatively loci can evolve allelic effects in opposition to their epistatic coefficients to reduce the phenotypic effects of new mutations. Figure 3 shows the relationship between average allelic effects and average epistatic coefficients in a small population ( N =128) in which large mutational variances evolve, and in a large population ( N =2,048) in which small mutational variances evolve. In the small population, we see a very weak, non-significant negative relationship between average allelic effects and average epistatic coefficients. However, in the large population, we see a strong and highly significant negative relationship. Thus, in the large population, loci with negative epistatic effects on average tend to have positive allelic effects and loci with positive epistatic effects tend to evolve negative allelic effects, with the consequence that the reference effects of most new mutations are largely counteracted by their opposing epistatic effects. This masking process due to opposing reference and epistatic effects is more important in larger populations than smaller populations, resulting in a negative relationship between mutational variances and population size. In Fig. 3 , for the sake of simplicity, we address only the evolution of the mutational variance at one trait, but the evolution of mutational covariances arises from similar processes. In short, the mutational architecture evolves as a consequence of the quantitative trait loci evolving allelic effects that interact with their epistatic coefficients according to the current regime of selection and drift. Figure 3: Epistasis allows the mutational variance to evolve as function of population size. The average allelic effect can evolve to be correlated with the average epistatic coefficient, and the strength of this relationship varies with population size. These data are from 20 independent simulation runs using our core parameter set, except with only 10 quantitative trait loci. In addition, we allow only within-trait epistasis affecting trait one and no epistasis involving trait two, with population sizes of ( a ) N =128 and ( b ) N =2,048. Each point represents a single quantitative trait locus. The x axis shows the magnitude of epistasis (mean epistatic effect of a locus, averaged across all of its epistatic coefficients), and the y axis presents the mean allelic effect (or reference effect) of alleles at the corresponding locus, averaged across all alleles segregating at the locus. In small populations, large mutational variances are maintained by the evolution of a large range in allelic effects; we see a slightly negative but non-significant relationship between epistatic coefficients and allelic effects (linear regression, N =200, R 2 =0.01, P =0.09). In large populations ( b ), which evolve lower mutational variances than small populations, we see a much smaller range in allelic effects and these effects show a strong negative relationship with the mean epistatic coefficients across loci (linear regression, N =200, R 2 =0.22, P <<0.0001). Thus, the allelic effects of a particular locus tend to evolve values that are largely counteracted by the epistatic effects of the locus in question. This figure is concerned with the evolution of the mutational variance, but a similar effect explains the evolution of mutational covariances. Full size image One other consequence of the evolution of the mutational architecture under epistasis is that the alignment of the M -matrix with the G -matrix will tend to strengthen any additive genetic correlations that exist in the population ( Tables 2 and 3 ). Except under very strong epistasis or large population size and strong epistasis, the majority of genetic variance arising from epistasis is additive ( Tables 2 and 3 ; Supplementary Table 3 ), which means that this genetic variance can contribute to a response to selection. Indeed, our results indicate that a mutational architecture evolving under epistasis can enhance a population’s ability to respond to selection. For instance, in small populations with very high mutational variances (caused by epistasis), we see a stronger response to selection compared with larger populations ( Supplementary Table 3 ). Much of the genetic variance in the smaller population is attributable to the large mutational variance, which is a product of the evolution of the mutational architecture made possible by epistasis. However, the majority of the genetic variance is nonetheless additive (compare V A with V G in Supplementary Table 3 ), and therefore available for natural selection. Similarly, the genetic covariance, which is strengthened by the alignment of the G -matrix and M -matrix, is mainly additive genetic in nature and thus produces a correlated response to selection ( Supplementary Table 3 ). Evolution of the M -matrix and triple alignment of the type we describe here occurs under almost all parameter combinations. Regardless of the strength of epistasis ( Table 2 ), population size ( Table 3 ), mutational variance of reference effects ( Supplementary Table 4 ) or strength of stabilizing selection ( Supplementary Table 5 ), we see a tendency for the M -matrix to align with the selection surface, as evidenced by the evolution of a positive mutational correlation in the presence of positive correlational selection. However, we do observe that the evolution of the mutational correlation becomes less pronounced as mutations become sufficiently rare ( Supplementary Table 6 ). Our analysis of the two-trait version of the multilinear model of epistasis provides several important insights into the evolution of the genetic variance of quantitative traits. The first key insight is that epistasis allows the evolution of mutational effects and in particular larger mutational effects and variances in smaller populations. These larger mutational variances, in turn, cause smaller populations to harbour greater amounts of additive genetic variance than larger populations, a counterintuitive result that is nevertheless consistent with the broader literature on the evolution of mutational effects and mutational robustness [32] , [33] , [34] , which is defined as the ability of an organism or trait to maintain its function despite the occurrence of novel mutations [33] . The second major insight from our model is that epistasis allows the mutational matrix to evolve towards alignment with the individual selection surface. As both the mutational matrix and the individual selection surface influence the shape and orientation of the G -matrix, we find that epistasis produces a situation of triple alignment, in which patterns of mutation, genetic variation and selection evolve towards a common orientation in phenotypic space. These results illuminate the potential importance of epistasis and the evolution of mutational effects in evolutionary processes. The most counterintuitive result in our study is that smaller populations evolve larger mutational variances than larger populations to such a degree that smaller populations tend to harbour greater levels of additive genetic variance in quantitative traits. This pattern likely arises from three main processes, one driven by epistasis and the other two arising from genetic drift. First, because epistasis is non-directional on average in our model (that is, positive and negative interactions potentially balance), mutational variance tends to increase in the absence of other evolutionary forces (see Methods). Second, the efficacy of stabilizing selection is lower in smaller populations, allowing these populations to maintain alleles with larger ‘reference’ effects, which can be thought of as the phenotypic effect the allele would have in the absence of epistasis. These larger reference effects in turn increase the absolute magnitude of epistatic contributions. In particular, large reference effects at some loci can be compensated for by large reference effects of opposite sign at other loci, thus leading to more compensatory evolution in small populations. For a seemingly similar observation in a different model, see the recent report from Rajon and Masel [35] . The third cause of a higher mutational variance in smaller populations is that stabilizing selection favours the evolution of smaller additive genetic variances [36] , a phenomenon that has been observed in other studies as an increase in mutational robustness in large populations [34] , [37] . As smaller populations tend to have their phenotypic means displaced away from the bivariate optimum by the action of genetic drift, they experience larger absolute forces of directional selection, which favors an increase in additive genetic variation [38] , and less stabilizing selection compared with larger populations. Therefore, the evolution of mutational robustness is less effective in the smaller populations. Together, these factors produce large mutational and additive genetic variances in small populations. Another possibility is that multiple quasi-stable equilibria exist in our simulated populations, a phenomenon that has been observed in other studies of the multilinear model of epistasis [26] , and that genetic drift allows smaller populations to shift between these equilibria more often than larger populations [39] . Such a scenario could also produce an increase in genetic variance and mutational variances in the small populations. Regardless, despite the fact that selection is less efficient in small populations due to the effects of genetic drift, our results show that the combined action of drift and selection can allow these small populations to maintain large mutational variances. Thus, these conflicting evolutionary pressures combine to produce a negative correlation between effective population size and mutational variances, and we see a pronounced manifestation of this expectation in our results ( Table 3 ). Our analysis of the evolution of the orientation of the mutational matrix extends previous work, which focused exclusively on the evolution of the mutational correlation. When the mutational correlation is treated as a quantitative trait in an additive model, it has a tendency to evolve towards alignment with the selection surface [20] . However, a much more realistic way to model the evolution of the M -matrix is by using an explicit, general model of epistasis, as we have done here. Our results show that, indeed, the mutational correlation does evolve towards alignment with the selection surface, and more importantly, the mutational variances and covariances evolve in tandem to produce a mutational matrix nearly perfectly aligned with the selection surface. Under these circumstances, the selection surface and mutational matrix both influence the standing genetic variance in the population, which also results in triple alignment of the M -matrix, G -matrix and selection surface. This alignment scenario is important from an evolutionary standpoint, because constraints imposed by the M -matrix can be quite strong [18] , [19] , but here we see that these mutational constraints are shaped in part by natural selection. Triple alignment means that new mutations entering the population will tend to fall along the ridge of the selection surface, if there is one, thus mitigating their deleterious impacts. Furthermore, triple alignment will facilitate evolution along both genetic and selective lines of least resistance [40] , [41] . Thus, the evolution of robustness and of evolvability occur simultaneously in our model [33] , [42] , [43] . Our study has several limitations that offer fodder for future work on how epistasis affects multivariate trait evolution. Importantly, we follow the convention of other individual-based studies of quantitative genetic phenomena, including epistasis, and use unrealistically high per-locus mutation rates. Although this rate inflation is likely to facilitate the evolution of genetic architecture [34] , this device is necessary because realistic per-locus mutation rates in such simulations tend to produce unrealistically low levels of additive genetic variance. For instance, with mutation rates of the order of 10 −6 or 10 −7 , our populations lose all genetic variation and all interesting evolutionary phenomena cease to occur. This result illustrates that we still do not fully understand the mechanisms maintaining genetic variation in natural populations, but it also represents a real constraint for the type of model we employ here [36] . It is worth noting, however, that our mutation rates are much more realistic than those used in some univariate studies of the multilinear model. Le Rouzic et al. [30] , for instance, employed a per-locus mutation rate of 0.01, arguing that the mutation rate has little effect on the qualitative dynamics of the system beyond affecting the timescale of evolution [44] , [45] . In addition, our model typically focused on quantitative traits determined by a small number of loci, typically 20, due to computational constraints. Actual traits in living systems may be affected by hundreds or thousands of loci, which would give them a much larger mutational footprint than the traits considered here. Moreover, if quantitative traits are sometimes affected by suites of physically linked genes, then mutations at these supergenes could occur more frequently than they would occur for any single gene in the genome. These sorts of tightly linked gene clusters are appropriately simulated by the type of model we used here, where each simulated locus could be interpreted as a group of physically linked genes affecting the phenotype. Regardless, progress in reconciling simulation-based models and real data will require additional data on the genetic details of multivariate, quantitative phenotypes. Our results also show that the type of epistasis influences the evolution of mutational architecture. Most of our simulations allow all possible pairwise epistatic effects. However, in our model all loci are pleiotropic, meaning each locus has an effect on trait one and an effect on trait two, so epistatic effects can potentially occur within or between trait effects across loci. If only within-trait effects are allowed (for example, the trait-one effect at one locus interacts with the trait-one effect at another locus to affect only the trait-one phenotype), then the mutational correlation cannot evolve ( Supplementary Table 7 ). Thus, the alignment of the M -matrix with the selection surface requires at least some between trait epistasis. Recent empirical studies indicate that this type of epistasis, necessary for the evolution of mutational covariances, does exist in natural populations. This type of epistasis has been termed ‘differential epistasis’ by Cheverud et al. [46] and has been shown to occur for morphological and physiological traits in mice [24] , [25] , [47] . The results of the present model should provide a foundation for studies involving more realistic assumptions, and several obvious directions for future studies emerge from our results. For instance, our model ignores complications such as dominance, directional epistasis and higher-order epistasis, all of which can influence the evolution of the mutational architecture [29] , [48] . We also allow all pairwise epistatic interactions among loci, whereas the genetic architectures of actual traits are probably determined by gene networks with far fewer epistatic interactions. Furthermore, we constrain the epistatic parameters to remain constant within a simulation run, a feature that we retain from the univariate version of the multilinear model. However, in actual biological systems, the strengths of epistatic interactions among loci may evolve. A model with evolving epistatic coefficients would require assumptions about the genetic basis and inheritance of epistatic effects and is well beyond the scope of the model we present here, but such a model could be very enlightening with respect to the evolution of mutational and genetic architectures of complex traits. In summary, the application of the multilinear model of epistasis to a two-trait phenotype results in several startling insights into the evolutionary process. The most important insight is that natural selection, embodied by the individual selection surface, causes mutational architectures to evolve in an adaptive way. This result contradicts the simplistic view of mutation presented in most texts in which mutation is claimed to be random with respect to adaptation. Our results reinforce and extend the results of other studies that have addressed various aspects of the evolution of the mutational architecture by exploring the effects of epistasis in the univariate case [28] , [29] , [30] , [31] , [39] , by examining the evolution of mutational correlations [20] , [47] , and by addressing the effects of phenotypic plasticity on the evolution of mutational processes [49] . Our approach is unique in that we allow the mutational variances and covariance to evolve simultaneously, and our results show a striking pattern of three-way alignment across levels of biological organization. In particular, the M -matrix, which describes the distribution of mutational effects entering the population, evolves to align with the individual selection surface. This alignment increases mutational robustness in the sense that it is expected to reduce the fitness impacts of novel mutations [32] , [34] . In turn, the G -matrix, which describes the standing levels of additive genetic variance in the population, evolves to align with both the M -matrix and the selection surface. This three-way alignment of mutation, genetic variation and selection is significant for a number of reasons. First, the mutational architecture of traits should not be seen as something that is independent of natural selection. Rather, the mutational architecture is partially a product of natural selection [50] . Second, the evolution of the M -matrix will tend to reinforce any genetic correlations produced by selection, and this reinforcement increases the efficacy of correlated responses to selection, which determine evolutionary trajectories in phenotypic space. Finally, the extent of alignment between the mutational architecture and the selection surface will influence the fitness effects of new mutations. Stronger alignment reduces the deleterious impacts of new mutations. In general, our results suggest that the already impressive forces of natural selection may extend to the very roots of the evolutionary process by shaping the nature of variation that enters populations as a consequence of novel mutations. The multivariate multilinear model Our Monte Carlo simulation is an extension of the models used by Jones et al. [18] , [19] , [20] to study the evolution of additive genetic variances and covariances in sexually reproducing populations. These models explicitly simulate all individuals in the population. Every individual has a two-trait phenotype determined by its genotype and random environmental effects. In the original models, all loci are assumed to be additive, so an individual’s genetic value is determined by simply summing across all alleles at all loci. As in the original model, all loci are assumed to be pleiotropic, so each allele has an effect on both traits and both effects for a particular allele are inherited together. The most important difference between the present model and previous models is the addition of epistasis. Our implementation of epistasis follows the multilinear model [28] , which has been used successfully to study the effects of epistasis on a univariate phenotype [29] , [30] , [31] . The addition of epistasis to the model changes the way a multilocus genotype is converted into a phenotype. The multilinear model simply extends the additive model by specifying additional terms, which describe the effects of epistasis. Thus, in the univariate multilinear model, the phenotype is given by where X is the individual’s genotypic value for the quantitative trait, ξ 0 is the value of an arbitrary reference genotype, which for our model with a stationary intermediate optimum can be assumed to be zero, y ( i ) is the reference effect of an individual’s genotype at locus i (the two allelic values in the diploid organism are summed to obtain the genotype’s reference effect) and ε ( i , j ) is an epistatic coefficient, which determines the nature of the interaction between locus i and locus j . Clearly, if all epistatic coefficients are zero, then this model reduces to a strictly additive model and the reference effects correspond to additive effects. This description of the multilinear model includes only pairwise interactions. In principle, higher-order interactions can be included in the model, but in the present study we allow only pairwise interactions between loci. The multiple trait version of this multilinear model requires additional notation and additional epistatic terms. In the present paper, we restrict attention to the two-trait case, which is simple enough to understand yet complex enough to capture the essence of the evolution of the multivariate phenotype. In our model, every locus is potentially pleiotropic, in the sense that it has a reference effect on both traits. In addition, every locus is potentially epistatic, as specified by the multilinear model. In this model, then, every individual has two genotypic values, one for each trait, specified by where a X is an individual’s genotypic value for trait a , and a ξ 0 is the value of the reference genotype, which will be zero for our analysis. As in the univariate case, a y ( i ) is the individual’s reference genotypic value on trait a at locus i , and in the absence of epistasis, this value would be the additive effect of the locus. The final summation term represents the epistatic interactions among loci, where abc ε ( i,j ) gives the epistatic effect on trait a of the interaction between the effects of locus i on trait b and locus j on trait c . We assume that no locus interacts with itself, so abc ε ( i,i ) =0 and that interactions are symmetric in the sense that abc ε ( i,j ) = acb ε ( j,i ) . Each epistatic term is simply the product of the relevant epistatic coefficient and the reference effects at the two interacting loci. However, this model allows the reference effects of the two loci on one trait to affect an individual’s genotypic value at another trait, so the model is general, and most forms of epistasis can be represented as special cases of this multivariate multilinear model. Equation (2) allows us to calculate an individual’s genotypic value across all loci at both traits, taking into account all possible pairwise epistatic interactions. We simulate environmental variance by drawing a value from a normal distribution with a mean of zero and a variance of one independently for each trait. These environmental effects are added to the genotypic values to determine an individual’s phenotypic value for each quantitative trait. The life cycle: mating, recombination and mutation Each generation of the simulated life cycle begins with the adults of the previous generation mating and producing zygotes. The epistasis model employs a mating system in which each female mates with exactly two males and produces a total of four offspring, two from each father. Mates are chosen at random, and individual males can mate as many times as they are chosen. This breeding design facilitates the estimation of quantitative genetic values, as described below. Alleles are inherited in a Mendelian fashion, and we assume that all loci are physically unlinked. Each gamete contributing to a zygote has a probability of nμ of carrying a new mutation, where n is the number of loci affecting the quantitative traits and μ is the per-locus mutation rate. Recalling that each locus affects both quantitative traits, we draw mutational effects at random from a bivariate normal distribution with mutational variances of (for trait one) and (for trait two) and a mutational correlation specified by r μ . These mutational effects are then added to the existing reference effects of the allele undergoing the mutation. Hence, each time a mutation occurs, it alters the pleiotropic allele’s effects on both traits. The changes are at the level of reference effects, which will be additive effects if all the epistatic parameters are zero. However, in the presence of epistasis, changes in reference effects do not necessarily translate directly into changes in additive effects. Even though the epistatic coefficients remain constant throughout a simulation run, the epistatic interactions can evolve as the allelic effects present at various loci change over time. As the epistatic interactions also determine the mapping of reference effects to the genotypic value of an individual, this model allows the M -matrix, which summarizes the distribution of new mutations entering the population, to evolve as well. The life cycle: selection We impose selection by assuming an individual selection surface with the shape of a bivariate Gaussian function. Assuming z is a vector of an individual’s phenotypic values at the traits under consideration, the probability of surviving selection is where θ is a vector of trait optima, T represents matrix transposition and ω is a matrix that describes the shape of the selection surface. In our two-trait case, ω is a symmetric 2 × 2 matrix with diagonal elements, analogous to variances, indicating the strength of stabilizing selection on each trait. Smaller values result in a steeper surface with stronger stabilizing selection. The off-diagonal element, analogous to the covariance, indicates the strength of correlational selection, and can be conveniently summarized as the selectional correlation, r ω , with larger absolute values corresponding to stronger correlational selection (see below). We impose viability selection by choosing a uniformly distributed pseudorandom number between 0 and 1 for each individual. If the number is less than W ( z ), then the individual survives to the next phase of the life cycle, population regulation. The life cycle: population regulation In this evolutionary model, we assume that a population is near its carrying capacity, K . We restrict attention to cases in which the population invariably produces more than K offspring, and we impose population regulation by choosing K individuals at random from the survivors of selection. We also impose an equal sex ratio on these adults. These individuals are the adults of the new generation, and they will go on to mate as described above to produce the next generation of progeny. Important parameter values In this model, we restrict attention to a population evolving in response to a stationary individual selection surface. Thus, genetic drift and stabilizing selection are the main sources of evolutionary change. Some directional selection occurs when drift moves the population away from the bivariate optimum, and this directional selection moves the population back toward the optimum. In the present analysis, we explore a large swath of parameter space, and we report results from the most important parameters. An exhaustive exploration of parameter space is intractable for this sort of model, so we start with a core set of parameter values and examine how deviations from this core set affect evolutionary dynamics. The core parameter set is given in Table 1 . Several of these parameters require some explanation. As noted above, the parameters describing the selection surface, ω , whose elements are ω 11 , ω 22 and ω 12 , are critically important because they determine the strength of selection and the extent to which correlational selection acts on the population. For convenience, we use the selectional correlation ( r ω ) rather than ω 12 , because r ω , which is constrained to fall between −1 and 1, is more conceptually understandable. Of course, r ω is simply , so the conversion between the selectional correlation and the selectional covariance is trivial. The mutational variances ( ) and mutational correlation ( r μ ) for reference effects determines the distribution of new mutations entering the population. Epistasis can cause the reference effects to be only loosely connected to the effects of the mutation on the genotype, so we specify the latter as the M -matrix (see below). The M -matrix is thus a variable (of considerable interest) in this model rather than a parameter, whereas the effects of mutations on the reference effects of alleles are true parameters that can be specified and remain constant for a given simulation run. As we are interested in the tendency for epistasis to generate mutational correlations, we use a value of zero for the mutational correlation of reference effects ( r μ ). Another feature of the epistasis model is that there are many epistatic coefficients. For instance, in a single-trait multilinear model, there will be a total of n ( n −1)/2 such coefficients, where n is the number of loci. In the two-trait multilinear model, there are six times as many coefficients, because all interactions between reference effects within and between traits must be considered. Thus, a model with 20 loci has a total of 1140 unique epistatic coefficients. The only feasible way to model epistasis, then, is to draw these coefficients from a distribution. We draw them from a normal distribution with a mean of zero and a variance of . This approach allows a mixture of positive and negative epistasis. One key aspect of this model is that the epistatic parameters are set at the beginning of each independent simulation run, and they do not change during the run. As the epistatic coefficients remain constant, the epistatic effects evolve as a consequence of changes in the reference effects of loci, which do evolve as a consequence of mutation, drift and selection. The other parameters listed in Table 1 also remain constant throughout a particular simulation run. Evolution of mutational effects We show for the univariate case that the mutational variance will increase in the absence of other evolutionary forces if there is no directional epistasis, that is, if E [ ε ]=0, as assumed throughout this paper. Consider just two loci. Then, by equation (1), the effect of a mutation of size α at the first locus is where we write ε = ε (1,2) . As E [ α ]=0, also E [Δ m ]=0. Taking expectations with respect to mutational effects, epistasis parameters and locus effects, the variance of mutational effects becomes where we used pairwise independence of α , ε and locus effects. Now, the assumption E [ ε ]=0 yields However, at each particular locus mutational variances may increase or decrease, depending on the particular choice of epistatic parameters. Statistical and estimation issues The addition of epistasis to our model carries with it a number of challenges regarding the estimation of variables of interest. In this study, we are interested in the distribution of total and additive genetic variance in the population at any given time, and we are also keenly interested in the evolution of the M -matrix, which serves as the central source of motivation of this study. We represent the elements of the M -matrix as M 11 , M 22 and M 12 , and we also specify the mutational correlation as r M (which is equal to ). We estimate the genetic variance components by building a half-sib breeding design into the model. By having each simulated female mate twice, we generate a number of half-sib families equal to the number of females in the population. The analysis of this breeding design can be accomplished through a standard analysis of variance approach [51] . Our population lacks dominance, so the total genetic variance can be partitioned into parts arising from additive genetic variance and additive-by-additive epistatic variance. Even when epistatic effects are large, much of the genetic variance arising from the epistatic terms in equation (2) is additive and thus contributes to parent–offspring resemblance. The M -matrix is prohibitively difficult to estimate analytically, due to the many epistatic interactions and the possible presence of linkage disequilibrium among loci, so we use an empirical approach to determine the distribution of mutational effects. Every 100 or 200 generations, we make a copy of all progeny produced and induce individual mutations 50 times per locus for each individual. After each single-locus mutation, we refigure each individual’s genotypic value for the two traits, as described in equation (2), and compare this new genotypic value to the value before mutation. The individual’s genotype is then set back to its original value before the next mutation. The change in the genotypic value is the effect of the mutation, and we use this approach to compile a distribution for each locus separately. In most cases, we report the average M -matrix, which we calculate as the mean mutational variances and mutational correlation across loci. For each simulation run, we start with an initial population of adults with population size ( N ) equal to the carrying capacity ( K ), and indeed N = K for the duration of each run. Each locus starts with five equally frequent alleles with allelic effects drawn from a bivariate normal distribution with a mean of zero, s.d. of the corresponding mutational s.d. divided by the number of loci, and covariance of zero. This initial population is then permitted to evolve for a period of 5,000 generations to reach a state of quasi-equilibrium between genetic drift, selection and mutation. These initial generations are followed by 5,000 experimental generations during which we calculate values of interest. For each combination of parameter values, we typically conduct 20 independent simulation runs. Variables are often averaged across generations within a run and then these means are averaged across runs to give the values we report. How to cite this article: Jones, A. G. et al. Epistasis and natural selection shape the mutational architecture of complex traits. Nat. Commun. 5:3709 doi: 10.1038/ncomms4709 (2014).